Ordinary percolation with discontinuous transitions Percolation on a one-dimensional lattice and fractals, such as the Sierpinski gasket, is typically considered to be trivial, because they percolate only at full bond density. By dressing up such lattices with small-world bonds, a novel percolation transition with explosive cluster growth can emerge at a non-trivial critical point. There, the usual order parameter, describing the probability of any node to be part of the largest cluster, jumps instantly to a finite value. Here we provide a simple example in the form of a small-world network consisting of a one-dimensional lattice which, when combined with a hierarchy of long-range bonds, reveals many features of this transition in a mathematically rigorous manner. The percolation properties [1] of networks are of significant interest—without percolation, any large-scale transport or communication through the network ceases. Much research has been dedicated to the understanding of percolation on randomly grown, complex networks [2] . Yet, the engineering of artificial networks with well-controlled features seems desirable. Indeed, there has been considerable interest in the properties of spatial networks, linking real-world geometry with small-world effects [3] , [4] , [5] . In particular, networks possessing hierarchical features [4] , [6] , [7] , [8] , [9] , [10] relate to actual transport systems such as for air travel, routers and social interactions. Certain hierarchical networks, with a self-similar structure, have been shown to exhibit novel features [8] , [11] , [12] , [13] , [14] , [15] . To these, we add here an unprecedented discontinuous transition in the formation of an extensive cluster for ordinary, random-bond addition. Such an extensive cluster is said to percolate, as it contains a finite fraction of all nodes. Remarkably, this discontinuous transition can be derived 'exactly' with recursive methods, as shown below. For a random network that allows bonds between any pair of nodes, the possibility of a discontinuous ('explosive') percolation transition has recently attracted considerable attention [16] , [17] , [18] , [19] , [20] , [21] , [22] , [23] , [24] , [25] , [26] , [27] , [28] . Such a transition raises the prospect that a minute increase in the bond density p of a network can suddenly make a large fraction of all nodes accessible, for instance, for the spreading of a contagion [29] . Yet, all proposed mechanisms for such a transition require 'correlated' bond additions [16] . Although further simulations of the dynamics of such correlated cluster formation [21] , [22] , [23] , [24] , [25] , [26] , [27] , [28] seemed to support the existence of a discontinuity, evidence against it [17] , [18] , [19] , [20] finally mounted into a general proof of the impossibility of explosive percolation for any of the proposed mechanisms [30] . In contrast to these efforts, we study ordinary (uncorrelated) bond additions, but on networks with a recursive, hierarchical structure to induce such an explosive percolation dynamics. Understanding of explosive cluster formation will be significantly advanced when the discontinuity can be studied rigorously by simply adding bonds randomly to these networks. Probability of a spanning cluster In our discussion, we focus on a simple example of a hierarchical network that is shown in Fig. 1 . In its hierarchical construction, networks from preceding generations are merged for successive generations for ever larger networks. The probability for an end-to-end path of the most elementary network at n =0, a single bond, is T n =0 = p . By merging two networks of generation n side-by-side and adding a long-range bond to obtain a network of generation n +1, we recursively determine the probability T n +1 . This analysis is but one example of the real-space renormalization group [31] . 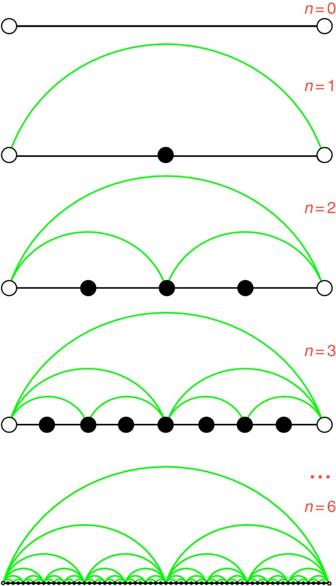Figure 1: Recursive generation of a hierarchical network. (The network is displayed at full bond density,p=1.) In (n=0)-th generation, the network consists of a single bond between two endnodes (open circles). The probability for an end-to-end path is obviouslyTn= 0=p. In successive generations,n+ 1= 1,2,..., two sub-networks from the previous generationnare merged together with the endpoints connected by a new long-range bond (shaded arcs). There is an end-to-end path with probabilityTn+ 1, if either the new long-range bond exists (probabilityp, irrespective ofTn) or both previous sub-networks are present (probability (1−p)T2n), leading to equation (1). In each generationnthe network hasN= 2n+ 1 nodes andE= 2n+1− 1 bonds for an average degree 2E/N~ 4 for largen. Figure 1: Recursive generation of a hierarchical network. (The network is displayed at full bond density, p =1.) In ( n =0)-th generation, the network consists of a single bond between two endnodes (open circles). The probability for an end-to-end path is obviously T n = 0 = p . In successive generations, n + 1= 1,2,..., two sub-networks from the previous generation n are merged together with the endpoints connected by a new long-range bond (shaded arcs). There is an end-to-end path with probability T n + 1 , if either the new long-range bond exists (probability p , irrespective of T n ) or both previous sub-networks are present (probability (1− p ) T 2 n ), leading to equation (1). In each generation n the network has N = 2 n + 1 nodes and E = 2 n +1 − 1 bonds for an average degree 2 E / N ~ 4 for large n . Full size image The probabilities for an end-to-end path satisfy the recursion as is explained in Fig. 1 . In the limit of infinitely large networks, we obtain for any p , the probability for such an end-to-end connection, , from the stationary solutions of equation (1), called 'fixed points'. Setting in equation (1) yields a horizontal line of fixed points T * ≡1 for all p , as well as arising line of fixed points, Both lines intersect at p = 1 / 2. Further analysis shows [11] that equation (2) is the stable solution for all 0 < p < 1/2 that describes the actual behaviour of large networks. That is, very large networks possess an end-to-end connection with a finite probability approaching 0 < T * ( p ) < 1. However, for 1/2 ⩽ p ⩽ 1, the horizontal line is the only physical and stable solution such that a connection exists with certainty, T * =1. Origin of the percolation transition The phenomenology of percolation on hierarchical networks is quite distinct from that of lattices [11] , [12] , [13] , [14] . Specifically, on a lattice both, an end-to-end path and an extensive cluster, arise with certainty above the same critical bond density p c . Each node attains a finite probability P ∞ ( p > p c ) > 0 to be connected to the spanning cluster. In contrast, hierarchical networks may have two transitions at a lower and an upper bond density, p l < p u . Below the lower transition p l , all clusters remain finite and no end-to-end paths exists. Above the upper transition p u , there is an extensive cluster and a certain end-to-end path, as on any lattice. But, both transitions delimit an interval p ∈ ( p l , p u ) that contains fractal (sub-extensive) clusters with a finite probability T * for an end-to-end path, as given by equation (2). These clusters each harbour a vanishing fraction of all nodes; however, they diverge in size with N Ψ , defining a new fractal exponent 0 ⩽ Ψ ( p ) < 1 [13] . Accordingly, the order parameter [1] , [31] P ∞ becomes non-zero only at p u , making it the thermodynamically correct transition point, p c = p u . In the present network, it is p l =0 and p u = 1/2; more elaborate networks with exact but non-trivial p l and p u are discussed elsewhere [11] . We note that the simultaneous emergence of an extensive cluster with end-to-end paths seems to be special for 'flat' geometries. Hierarchical networks possess what is called a hyperbolic geometry [10] , for which most nodes are close to the periphery, similar to a tree, with many root-to-end paths. Correspondingly, parabolic networks would be very prone to clustering in the bulk with few paths to any peripheral node, that is, an extensive cluster would emerge before paths that access the periphery arise. Construction of the order parameter To reveal the nature of the transition, the probability T * ( p ) alone provides insufficient information. In addition, we have to derive the average size 〈 s max 〉 n of the largest cluster and as the proper order parameter [1] from cluster-generating functions. Thus, we introduce two basic quantities: the probability t i ( n ) ( p ) that both endnodes are connected to the same cluster of size i , and the probability s i,j ( n ) ( p ) that the left endnode is connected to a cluster of size i and the right endnote to a different cluster of size j . The corresponding generating functions, to provide the average cluster size, are defined as and are depicted in Fig. 2 . T n ( x ) represents clusters with an effective bond between the endnodes whereas S n ( x , y ) represents those that fail to provide such a bond. The following steps, while subtle, only entail elementary manipulations that result in three coupled but linear recursions. Although we provide enough details here to reproduce the intermediate steps in a few lines, we have implemented those steps also as a Mathematica script provided in the Supplementary Software . Therein lies the advantage of our present example: The discontinuity can be obtained exactly and with ease. 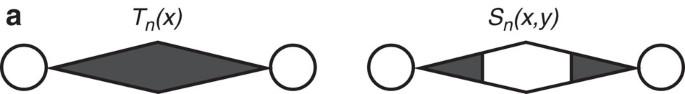Figure 2: Diagramatic defintion of the generating functions. In the schematic for generating functions, the open circles represent the endnodes, shaded areas indicate clusters that either span (Tn) or do not span (Sn) between the endnodes. Clusters that do not reach an endnode are ignored. Figure 2: Diagramatic defintion of the generating functions. In the schematic for generating functions , the open circles represent the endnodes, shaded areas indicate clusters that either span ( T n ) or do not span ( S n ) between the endnodes. Clusters that do not reach an endnode are ignored. Full size image The recursion relations for these generating functions are obtained in Fig. 3 by considering all possible configurations on three nodes, similar to Fig. 1 but now also taking cluster sizes into account. For each configuration, the type of effective bond between each of the nodes is checked, see Fig. 2 , and these bonds are assigned a value T n ( x ) or S n ( x , y ), depending on the type of cluster each represents. As in Fig. 1 , small-world bonds are merely assigned the probability p or 1− p for being present or not. Marking the increment in cluster size, the inner node provides a factor of x or y for its adjacent cluster, or unity if it remains isolated. The contribution of each configuration to the next generation is the product of the weights of the three bonds and of the intermediate node; all eight of these are determined in Fig. 3 . From Fig. 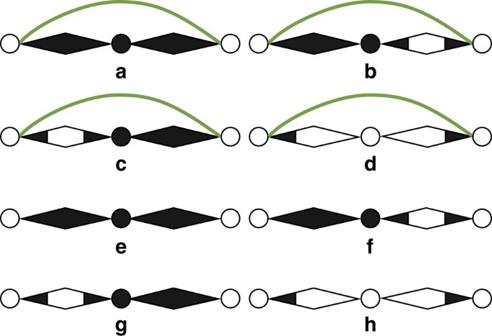Figure 3: Diagramatic evaluation of the generating functions. All diagrams contributing toin thenth real-space recursion group step are shown. The remaining endnodes (always-open circles) are not counted in the generating functions; the (black) connecting nodes increment the cluster size, accounted for by a factor ofxory. The contribution of each configuration is: (a), (b), (c), (d), (e), (f), (g), and (h). As tallied up in equations (6,7), configurations (a)–(e) span end-to-end and contribute toTn+1(x), while (f)-(h) do not span and contribute toSn+ 1(x, y). 3 , we read off the recursions Figure 3: Diagramatic evaluation of the generating functions. All diagrams contributing to in the n th real-space recursion group step are shown. The remaining endnodes (always-open circles) are not counted in the generating functions; the (black) connecting nodes increment the cluster size, accounted for by a factor of x or y . The contribution of each configuration is: ( a ) , ( b ) , ( c ) , ( d ) , ( e ) , ( f ) , ( g ) , and ( h ) . As tallied up in equations (6,7), configurations ( a )–( e ) span end-to-end and contribute to T n +1 ( x ), while ( f )-( h ) do not span and contribute to S n + 1 ( x, y ). Full size image initiated with . Naturally, both equations reduce to equation (1) for x = y = 1 where . The recursions in equations (6,7) contain more information than is needed here, and we simplify them in terms of functions of a single variable x . We define the functions Σ n ( x ) ≡ S n ( x,x ) and S n ( x ) ≡ S n ( x ,1) = S n (1, x ) that, combined into a more efficient vector notation V = [ T ,Σ, S ], lead to with a function-vector F of non-linear components As needed in equation (3), the mean size 〈 s max 〉 n of the cluster connected to the endnodes results from the first moment of the generating functions. These are obtained via their first derivative in x at x =1, for a network of size N = 2 n + 1 → ∞. Analysis of the recursions for the mean cluster size The mean size of the largest cluster, as needed in equation (3) to construct the order parameter, is obtained by Taylor-expanding equation (8) to first order in ɛ ≡ 1 − x → 0. To zeroth order, each component in equation (8) evaluated at x =1 reproduces equation (1) again. To order ɛ , we find an linear inhomogeneous recursion for , dropping the now-redundant argument x =1, with the Jacobian matrix and the inhomogeneity from differentiating for x explicitly In equations (12) and (13) we neglected the index n on and its components to simplify the presentation. They depend on n through . Since each network at n =0 only consists of endnodes, which are not counted, all clusters are initially empty, that is, . For large n at x =1, that is, near the fixed point , it is easy to show that the inhomogeneity in equation (11) is subdominant, leaving a linear homogeneous system with constant coefficient-matrix . The largest eigenvalue λ of this matrix provides the dominant contribution for each component of . We obtain λ between the transitions, , by applying equation (2) for T * in the matrix. Via equation (10), it is , which yields the fractal exponent The largest eigenvalue always remains , which implies that the order parameter P ∞ in equation (3) vanishes for . Above and at the transition, , it is T * =1 and equation (12) provides uniformly λ =2, as the largest eigenvalue (that is, Ψ ≡1), indicating percolation in form of an extensive cluster. For a continuous transition, . In contrast, equation (11) can be shown rigorously to provide a monotone increasing sequence for T n ′ , exactly at p = p c = 1/2 and for any p above (see Supplementary Software ). Therefore, the order parameter is positive definite even exactly at p = p c , as displayed in Fig. 4 . In fact, the continuity of P ∞ ( p ) is interrupted merely because T * ≡ 1 suddenly becomes an 'unstable' fixed point of equation (1) below p c . There, the stable branch transitions to equation (2) that lacks extensive clusters, Ψ < 1. Hence, it is the intersection of two stable branches of fixed points T * at p u that causes a discontinuous transition. Such intersections of lines of fixed points is generic in hierarchical networks [11] , whereas fixed points for percolation on lattices always remain 'isolated'. 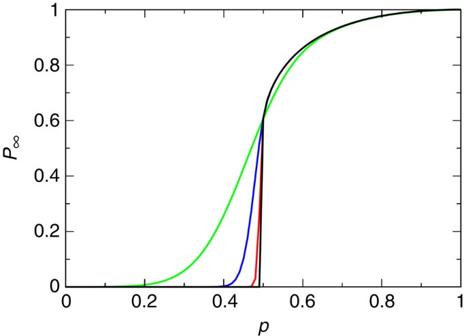Figure 4: Plot of the order parameterP∞(p) in equation (3). P∞(p) is evaluated aftern= 10kiterations of the recursions in equation (11) withk= 1,...,5,, displayed from left to right. This corresponds to system sizes of up tonodes. It evolves slowly into a discontinuity at. Convergence is slowest just belowpc, as finite-size corrections decay asfrom equation (14). Figure 4: Plot of the order parameter P ∞ ( p ) in equation (3). P ∞ ( p ) is evaluated after n = 10 k iterations of the recursions in equation (11) with k = 1,...,5,, displayed from left to right. This corresponds to system sizes of up to nodes. It evolves slowly into a discontinuity at . Convergence is slowest just below p c , as finite-size corrections decay as from equation (14). Full size image We have shown that a hierarchy of small-world bonds grafted onto a one-dimensional lattice can result in an explosive percolation transition, even if bonds are added sequentially in an uncorrelated manner. The discontinuous transitions found in hierarchical networks are unique as alternative models, based on correlated bond additions, have been proven to fail [30] . At this point, the precise conditions to be imposed on the hierarchy of long-range bonds for obtaining this transition are not entirely clear. However, in each example we have examined, the addition of small-world bonds converted an initially finitely ramified network into an infinitely ramified network to provide p c < 1, as several other networks demonstrate [11] . In a finitely ramified network, by definition [1] , the removal of just a finite number of bonds can separate off extensive clusters in the limit of large systems, N → ∞, resulting in p c = 1. In contrast, studies of hierarchical systems with small-world bonds imposed on a priori infinitely ramified 2d-lattices [11] , [12] , [14] seem to result in infinite-order transitions instead, which have been observed in many other networks [32] . How to cite this article: Boettcher, S. et al . Ordinary percolation with discontinuous transitions. Nat. Commun. 3:787 doi: 10.1038/ncomms1774 (2012).